Loss of beta2-integrin-mediated cytoskeletal linkage reprogrammes dendritic cells to a mature migratory phenotype The actin cytoskeleton has been reported to restrict signalling in resting immune cells. Beta2-integrins, which mediate adhesion and cytoskeletal organization, are emerging as negative regulators of myeloid cell-mediated immune responses, but the molecular mechanisms involved are poorly understood. Here, we show that loss of the interaction between beta2-integrins and kindlin-3 abolishes the actin-linkage of integrins and the GM-CSF receptor in dendritic cells. This leads to increased GM-CSF receptor/Syk signalling, and to the induction of a transcriptional programme characteristic of mature, migratory dendritic cells, accumulation of migratory dendritic cells in lymphoid organs, and increased Th1 immune responses in vivo . We observe increased GM-CSF responses and increased survival in neutrophils where the interaction between integrin and the cytoskeleton is disrupted. Thus, ligand-reinforced beta2-integrin tail interactions restrict cytokine receptor signalling, survival, maturation and migration in myeloid cells and thereby contribute to immune homeostasis in vivo . Dendritic cells (DCs) function as the main antigen-presenting cells in the immune system. These cells are highly mobile and orchestrate immune responses by taking up antigen in the periphery before migrating to lymph nodes in both steady-state and inflammatory conditions, where antigen is presented to T cells. The maturation or differentiation state of the DC determines the outcome of the immune response, and DCs control the initiation of helper, cytolytic and regulatory T-cell responses in vivo . Beta2-integrin adhesion receptors are expressed in both T cells and DCs where they play strikingly different roles in immune regulation. In T cells, beta2-integrins and their regulation by talin and kindlin-3 are required for firm adhesion under conditions of shear flow, and therefore for T-cell trafficking into lymph nodes and inflammatory sites [1] , [2] , [3] , [4] . Talin (but not kindlin-3) is required for efficient T-cell activation in vitro and in vivo [1] , [2] , [5] . In DCs, beta2-integrins play a very different role, as they are not required for DC migration to lymph nodes in steady-state [6] . Instead, beta2-integrins have been described to restrict DC-mediated priming of T cells [7] , [8] , [9] and Th17 differentiation [10] , although the molecular mechanisms involved have remained unclear. Beta2-integrins have been reported to play a regulatory role in macrophages by restricting Toll-like receptor (TLR) signalling through pathways dependent on Syk and IL-10 (refs 11 , 12 ), but have also recently been reported to promote TLR4 signalling in endosomes in DCs and DC-mediated T-cell activation [13] . Therefore, both the roles of beta2-integrins in DC signalling and the molecular mechanisms involved in regulation of DC-mediated immune responses by beta2-integrins remain unclear. Integrins integrate the cell exterior to the actin cytoskeleton, and integrin activation and signalling is regulated by the binding of cytoplasmic proteins, such as talin and kindlin-3, to the beta2-integrin cytoplasmic domain [14] , [15] , [16] , [17] , [18] . Kindlin-3 is an essential integrin regulator that binds to the integrin beta-chain cytoplasmic tail through a membrane-distal NPXY domain [19] and a TTT-domain [1] . A deficiency in kindlin-3 causes leukocyte adhesion deficiency type III (LAD-III), a disorder where beta2- and beta3-integrins cannot mediate leukocyte and platelet adhesion. LAD-III patients have a similar phenotype to patients with beta2-integrin subunit mutations (LAD-I), in that they suffer recurrent infections, with the addition of severe bleeding due to loss of platelet adhesion [16] , [20] . Recently, the actin cytoskeleton has been implicated in restriction of signalling in resting immune cells, by causing compartmentalization of the plasma membrane and thereby restricting mobility of cell surface receptors and associated molecules [21] . Whether integrins, the main ‘integrators’ of cell exterior and actin cytoskeleton in cells, contribute to this process has remained unclear. Here, we show that in the absence of beta2-integrins or beta2-integrin-kindlin-3-mediated cytoskeletal organization, bone marrow-derived DCs (BMDCs) display loss of association of the GM-CSF receptor with the actin cytoskeleton, increased GM-CSF receptor signalling and a maturation phenotype characteristic of in vivo migratory DCs, which leads to increased Th1 priming. Our data reveal a novel function of ligand-reinforced beta2-integrin-tail interactions in the restriction of cytokine receptor signalling of myeloid cells, and of myeloid cell survival, maturation and migration in vivo. The integrin-kindlin link in DCs restricts T-cell activation To investigate beta2-integrin-mediated regulation of immune responses, we used a mouse model that has recently been described where the kindlin-3 binding site in the beta2-integrin cytoplasmic domain has been mutated (beta2 TTT/AAA integrin knock-in mice) [1] . We have previously investigated the activation of T cells from beta2 TTT/AAA integrin knock-in mice, using in vitro models and in vivo adoptive transfer systems with WT DCs to prime T-cell responses, and found knock-in T-cell activation to be normal [1] . To investigate the role of the integrin-kindlin-3 interaction in DC-mediated immune responses in vivo , beta2 TTT/AAA integrin knock-in mice were immunized with peptide antigen in complete Freund’s adjuvant (CFA) to induce T-cell activation by beta2 TTT/AAA integrin knock-in DCs. Strikingly, we found that the CD4 T-cell response generated in both the spleen and the draining (inguinal) lymph nodes of beta2 TTT/AAA integrin knock-in mice was elevated compared with WT mice ( Fig. 1a ). This result led us to investigate the phenotype of beta2 TTT/AAA integrin knock-in DCs. 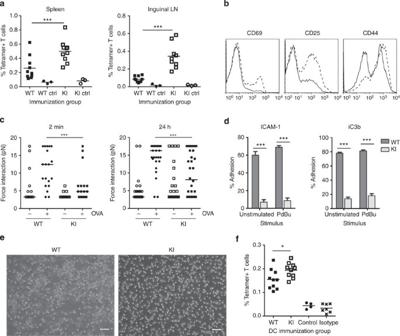Figure 1: The integrin-kindlin link in DCs restricts T-cell activationin vivo. (a) WT and knock-in (KI) mice were immunized subcutaneously with H19env peptide emulsified in CFA, and the T-cell response in the spleen and inguinal (draining) lymph nodes analysed using MHC class II tetramers 9d later. Each data point represents an individual mouse, with mean displayed, pooled from two independent experiments, with five mice per group per experiment. Control groups received no immunization. (b) WT or KI resting peptide-loaded BMDCs were cultured with CD4 OT-II T cellsin vitroat a ratio of 1:10. T-cell expression of CD69 (on day 1), CD25 (on day 2) and CD44 (on day 4) was analysed. Solid line—WT DCs, dashed line—KI DCs. Data are representative of N=4. (c) WT or KI BMDCs were pulsed with 1 mg ml−1OVA or left un-pulsed before addition of OVA-specific OT-II T cells. The force required to separate DCs and T cells after 2 min or 24 h of contact was determined. Each data point represents a single cell, with cells taken from two mice, and median indicated.P-values were calculated using the Mann–WhitneyU-test. (d) BMDC adhesion to ICAM-1 and iC3b was measured by static adhesion assay. N=4–7. Error bars indicate s.e.m. (e) BMDCs were imaged after 10 days of culture in GM-CSF. Images are representative of N=5. Scale bar, 100 μm. (f) WT or KI LPS-activated, peptide-loaded BMDCs were adoptively transferred into WT-recipient mice intravenously, and the T-cell response in the spleen measured 7 days later using MHC class II tetramers. Each data point indicates an individual mouse, with mean displayed. The control group received no adoptive transfer. Data are pooled from two independent experiments, with five mice per group in each experiment. In (a), (d) and (f) significant values were calculated using the Student’st-test. AllP-values are shown as <0.05*, <0.01**, <0.005***. Figure 1: The integrin-kindlin link in DCs restricts T-cell activation in vivo . ( a ) WT and knock-in (KI) mice were immunized subcutaneously with H19env peptide emulsified in CFA, and the T-cell response in the spleen and inguinal (draining) lymph nodes analysed using MHC class II tetramers 9d later. Each data point represents an individual mouse, with mean displayed, pooled from two independent experiments, with five mice per group per experiment. Control groups received no immunization. ( b ) WT or KI resting peptide-loaded BMDCs were cultured with CD4 OT-II T cells in vitro at a ratio of 1:10. T-cell expression of CD69 (on day 1), CD25 (on day 2) and CD44 (on day 4) was analysed. Solid line—WT DCs, dashed line—KI DCs. Data are representative of N=4. ( c ) WT or KI BMDCs were pulsed with 1 mg ml −1 OVA or left un-pulsed before addition of OVA-specific OT-II T cells. The force required to separate DCs and T cells after 2 min or 24 h of contact was determined. Each data point represents a single cell, with cells taken from two mice, and median indicated. P -values were calculated using the Mann–Whitney U -test. ( d ) BMDC adhesion to ICAM-1 and iC3b was measured by static adhesion assay. N=4–7. Error bars indicate s.e.m. ( e ) BMDCs were imaged after 10 days of culture in GM-CSF. Images are representative of N=5. Scale bar, 100 μm. ( f ) WT or KI LPS-activated, peptide-loaded BMDCs were adoptively transferred into WT-recipient mice intravenously, and the T-cell response in the spleen measured 7 days later using MHC class II tetramers. Each data point indicates an individual mouse, with mean displayed. The control group received no adoptive transfer. Data are pooled from two independent experiments, with five mice per group in each experiment. In ( a ), ( d ) and ( f ) significant values were calculated using the Student’s t -test. All P -values are shown as <0.05*, <0.01**, <0.005***. Full size image We assessed the T-cell priming ability of knock-in BMDCs in a co-culture system with TCR transgenic CD4 T cells specific for the ovalbumin (OVA) 323-339 peptide (OT-II T cells). Resting (non-TLR activated) peptide-loaded beta2 TTT/AAA -integrin knock-in DCs induced higher levels of OT-II T-cell activation in vitro , as measured by T-cell expression of the activation markers CD69, CD25 and CD44 ( Fig. 1b ). Using optical trapping, we show that knock-in DCs formed weaker antigen-dependent contacts with OT-II T cells, at both the initial contact (2 min) and at longer (24 h) contact times, compared with WT cells ( Fig. 1c ). This reduced adhesion strength is likely due to impaired binding of the integrin ligand ICAM-1 on the T-cell surface by DC beta2-integrins, as the kindlin–integrin interaction has been described to regulate integrin adhesion to ligands [1] . Indeed, knock-in DCs showed reduced binding to the beta2-integrin ligands ICAM-1 and iC3b ( Fig. 1d ), as well as to culture plates ( Fig. 1e ), demonstrating the general importance of beta2-integrin–kindlin-3 interactions in integrin-mediated cellular adhesion. As has been reported for other cell types carrying the TTT/AAA mutation [1] , surface expression of beta2-integrins was lower in knock-in DCs ( Supplementary Fig. 1A ), likely due to a deficiency in sorting nexin binding to the mutated integrin, leading to deficient integrin recycling from endosomes [22] . Indeed, treatment of cells with a lysosome inhibitor, bafilomycin, completely rescued the integrin surface expression defect in beta2 TTT/AAA integrin-expressing cells ( Supplementary Fig. 1B ). However, bafilomycin treatment did not rescue cell adhesion to ICAM-1 ( Supplementary Fig. 1C ), confirming that the defect in DC adhesion is due to impaired integrin function rather than a deficiency in integrin surface expression. Next we investigated CD4 T-cell activation in vivo using MHC class II tetramers following the adoptive transfer of either WT or knock-in LPS-activated peptide-loaded DCs into WT recipient mice. In this system, only the DCs carry the TTT/AAA mutation while all other cell types are WT. In agreement with the in vitro data, beta2 TTT/AAA -integrin knock-in DCs triggered a larger T-cell response in vivo in the spleen than WT DCs ( Fig. 1f ), although as this experiment used small amounts of adoptively transferred DC, which have to survive and migrate in the WT hosts, the CD4 T-cell response was not upregulated as much as in Fig. 1a , as expected. Taken together, these results suggest that beta2 TTT/AAA -integrin knock-in DCs are pre-disposed to activate T cells without TLR stimulation, driving elevated T-cell activation in vitro and in vivo , despite showing reduced adhesion to integrin ligands and forming weaker antigen-dependent contacts with T cells. Beta2-integrin knock-in DCs display elevated maturation Our results show that adhesion-deficient beta2 TTT/AAA -integrin knock-in DCs drive increased T-cell immune responses in vitro and in vivo . To further investigate the phenotype of knock-in BMDCs, expression of surface markers was analysed by flow cytometry. Surprisingly, expression of MHC class II and co-stimulatory molecules CD80, CD86 and CD40 was higher in GM-CSF-cultured, as well as LPS-activated, knock-in DCs compared with WT cells ( Fig. 2a,b ). Interestingly, expression of these markers showed a dose-dependent increase in response to GM-CSF ( Supplementary Fig. 2A ). Bafilomycin treatment of the knock-in DCs, which rescued cell surface expression of TTT/AAA integrins, did not inhibit these increased responses to GM-CSF ( Supplementary Fig. 1D ), demonstrating that the decreased surface expression of integrins in knock-in DCs was not responsible for their active phenotype. In terms of cytokine production by knock-in DCs, IL-12p40 was significantly increased with GM-CSF stimulation, while IL-12p40, IL-12p70, IL-10, IL-23p19, TNF-alpha and nitric oxide were elevated following LPS stimulation ( Fig. 2c and Supplementary Fig. 2B ), indicating that GM-CSF and TLR responses were elevated in knock-in cells. 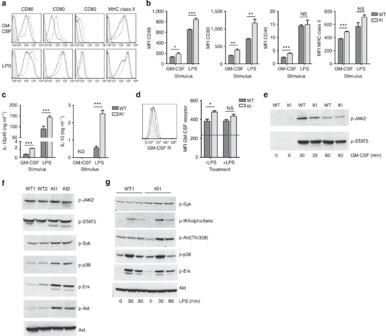Figure 2: Beta2-integrin knock-in DCs have elevated responsiveness to GM-CSF. (a) Expression of CD80, CD86, CD40 and MHC class II by WT (solid line) and KI (dashed line) BMDCs after 24 h stimulation with 10 ng ml−1GM-CSF or 100 ng ml−1LPS. Histograms are representative of N=4. Shaded line—isotype control. (b) Expression of activation markers by WT and KI BMDCs following 24 h stimulation with GM-CSF or LPS;N=4. (c) Cytokine production by WT and KI DCs was measured after 24 h stimulation with GM-CSF or LPS.N=3–5. ND=not detectable. (d) Surface expression of GM-CSF receptor by WT and KI BMDCs, showing representative histogram (WT solid line; KI dashed line; isotype control shaded line) and pooled dataN=3 (dashed line represents isotype control). (e) WT and KI BMDC were starved of GM-CSF for 60 min and then stimulated for the indicated times with 10 ng ml−1GM-CSF, and analysed for pJAK2 and pSTAT5 by western blotting. Representative of N=3. (f) WT and KI BMDCs were lysed following 3 h stimulation with fresh addition of 10 ng ml−1GM-CSF to DC cultures (without GM-CSF starvation), and analysed for phosphorylated (p-) signalling molecules or Akt (loading control) by western blotting. Data showN=2 and is representative of N=4. (g) WT and KI DCs were stimulated with 100 ng ml−1LPS for up to 60 min before lysis. Signalling molecules were analysed by western blotting. Data representN=3. All error bars show s.e.m. and significant values were calculated using the Student’st-test. AllP-values are shown as <0.05*, <0.01**, <0.005***. Figure 2: Beta2-integrin knock-in DCs have elevated responsiveness to GM-CSF. ( a ) Expression of CD80, CD86, CD40 and MHC class II by WT (solid line) and KI (dashed line) BMDCs after 24 h stimulation with 10 ng ml −1 GM-CSF or 100 ng ml −1 LPS. Histograms are representative of N=4. Shaded line—isotype control. ( b ) Expression of activation markers by WT and KI BMDCs following 24 h stimulation with GM-CSF or LPS; N =4. ( c ) Cytokine production by WT and KI DCs was measured after 24 h stimulation with GM-CSF or LPS. N =3–5. ND=not detectable. ( d ) Surface expression of GM-CSF receptor by WT and KI BMDCs, showing representative histogram (WT solid line; KI dashed line; isotype control shaded line) and pooled data N =3 (dashed line represents isotype control). ( e ) WT and KI BMDC were starved of GM-CSF for 60 min and then stimulated for the indicated times with 10 ng ml −1 GM-CSF, and analysed for pJAK2 and pSTAT5 by western blotting. Representative of N=3. ( f ) WT and KI BMDCs were lysed following 3 h stimulation with fresh addition of 10 ng ml −1 GM-CSF to DC cultures (without GM-CSF starvation), and analysed for phosphorylated (p-) signalling molecules or Akt (loading control) by western blotting. Data show N =2 and is representative of N=4. ( g ) WT and KI DCs were stimulated with 100 ng ml −1 LPS for up to 60 min before lysis. Signalling molecules were analysed by western blotting. Data represent N =3. All error bars show s.e.m. and significant values were calculated using the Student’s t -test. All P -values are shown as <0.05*, <0.01**, <0.005***. Full size image As cellular responses to GM-CSF were elevated in beta2 TTT/AAA integrin knock-in DCs, we went on to investigate GM-CSF signalling in knock-in BMDCs. Surface expression of the GM-CSF receptor was slightly increased in knock-in DCs compared with WT cells ( Fig. 2d ). The GM-CSF receptor signals through the JAK/STAT pathway leading to activation of further downstream pathways such as MAPK and Akt. Although initial JAK2/STAT5 activation after GM-CSF stimulation was similar in WT and KI cells ( Fig. 2e ), GM-CSF signalling was sustained in knock-in DCs, which displayed increased levels of p-MAPK, p-p38 and p-Akt downstream of JAK/STAT signalling at a 3-h time point after GM-CSF addition ( Fig. 2f ). Syk has been previously shown to be downstream of beta-common chain-containing cytokine receptor signalling [23] , and we found here that Syk signalling was also upregulated in beta2 TTT/AAA integrin-expressing cells downstream of the GM-CSF receptor ( Fig. 2f ). TLR (LPS) stimulation did not further increase Syk signalling in these cells, but LPS stimulation did result in upregulation of NFκB and Akt signalling in knock-in DCs, while levels of p-p38 and pErk after LPS stimulation were similar in WT and knock-in cells ( Fig. 2g ). These results demonstrate that GM-CSF (and TLR) signalling is upregulated in DCs where the kindlin-3-integrin link has been disrupted. Knock-in neutrophils show increased responsiveness to GM-CSF To investigate whether increased GM-CSF signalling was a general feature in the beta2 TTT/AAA integrin knock-in mice, we investigated neutrophil GM-CSF responses. Neutrophilia is a significant symptom in murine models with defects in adhesion molecules, including the recently developed beta2 TTT/AAA integrin knock-in mouse [1] , [24] , [25] , [26] , [27] . In addition to the previously reported increase in neutrophil numbers in the bloodstream of these mice [1] , we found neutrophil numbers in the bone marrow of beta2 TTT/AAA integrin knock-in mice to be significantly elevated compared with WT controls ( Supplementary Fig. 3A ). As GM-CSF is known to be vital for neutrophil survival [28] , we tested the survival capacity of WT and knock-in neutrophils in vitro . The results show significantly increased ex vivo survival of knock-in neutrophils, both in the absence of GM-CSF, likely reflecting continuing cellular responses to endogenous signals from their environment within tissues of the mice, and in the presence of GM-CSF ( Supplementary Fig. 3B ). Knock-in neutrophils also showed increased GM-CSF signalling ( Supplementary Fig. 3C ). These data demonstrate a more general role for beta2-integrins in the regulation of GM-CSF signalling in leukocytes. Knock-in bone marrow cells show elevated IL-3 response As the GM-CSF receptor shares the beta-common chain with the IL-3 and IL-5 cytokine receptors, we went on to investigate IL-3 responses in myeloid leukocytes. Myeloid leukocytes survived in culture without IL-3, but interestingly, beta2-integrin knock-in bone marrow myeloid cell proliferation in response to IL-3 was significantly increased compared with WT cells, with a greater effect seen at highest IL-3 concentrations (day 4 average MFIs for CFSE in KI cell cultures are 171 at 0.1 ng ml −1 IL-3; 135 at 1 ng ml −1 IL-3; 110 at 10 ng ml −1 IL-3), although the effects on survival were not very substantial ( Supplementary Fig. 3D ). These data indicate that beta2-integrins are especially important in the regulation of GM-CSF receptor (and TLR) signalling. In contrast, Flt3 ligand-cultivated DCs and M-CSF-cultured macrophages did not display increased activation responses ( Supplementary Fig. 4A,B ). Collectively, these results suggest that beta2 TTT/AAA integrin knock-in myeloid cells are more responsive to GM-CSF/IL-3 family of cytokines than WT cells. Beta2-integrin knock-in DCs have mature migratory phenotype Our data imply that maturation status is affected in adhesion-deficient beta2 TTT/AAA -integrin knock-in DCs. To investigate the global effects on gene transcription in these cells, we performed next-generation sequencing (RNAseq) from WT and beta2 TTT/AAA integrin knock-in BMDCs to map the transcriptomes. The data reveal that there were significant differences in gene expression between WT and knock-in DCs ( Fig. 3a,b and Supplementary Datasets 1-2 ). Co-stimulatory molecules CD86 and CD40 and cytokines such as IL-12 were confirmed to be upregulated on the transcriptional level in knock-in cells ( Fig. 3b ). Also, molecules involved in antigen presentation (MHC class II and CIITA), and in the JAK/STAT signalling (JAK2, STAT5, SOCS2) pathway were upregulated, while components involved in antigen uptake (Sort1, CD68, Stab1) were downregulated in knock-in cells ( Fig. 3b ), confirming that the maturation status was indeed affected in knock-in DCs. However, antigen uptake was not reduced in knock-in cells ( Fig. 3c ), indicating that the cells can still take up antigen, although they are in a more mature state. 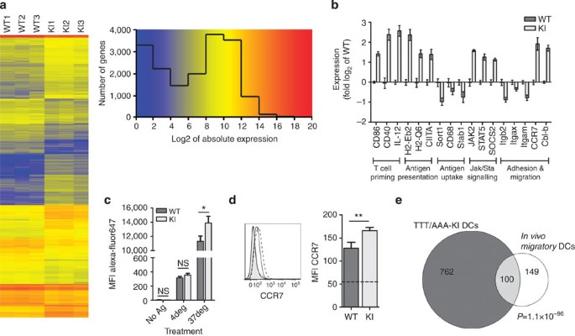Figure 3: Beta2-integrin knock-in DCs have a mature migratory phenotypein vitro. (a) Heat map of transcripts identified by RNAseq that show at least twofold differences in expression between WT and KI BMDCs;N=3. (b) Expression of biologically relevant genes in WT and KI BMDCs identified by RNAseq;N=3. (c) WT and KI BMDCs were incubated with 0.1 mg ml−1of OVA-alexa fluor 647 for 2.5 h at either 4 °C (4 deg) or 37 °C (37 deg). Antigen uptake was then measured by flow cytometry;N=7. (d) CCR7 expression by WT and KI BMDCs was determined by flow cytometry, with representative histogram (WT solid line; KI dashed line; isotype control shaded line) and pooled data fromN=3. (e) Venn diagram showing numbers and overlap of the gene expression profiles ofin vivomigratory DCs29and KI GM-CSF-cultured BMDCs. Significant values in (c,d) were calculated using the Student’st-test, and theP-value in (e) was calculated by Hypergeometric test. AllP-values are shown as <0.05*, <0.01**. Figure 3: Beta2-integrin knock-in DCs have a mature migratory phenotype in vitro . ( a ) Heat map of transcripts identified by RNAseq that show at least twofold differences in expression between WT and KI BMDCs; N =3. ( b ) Expression of biologically relevant genes in WT and KI BMDCs identified by RNAseq; N =3. ( c ) WT and KI BMDCs were incubated with 0.1 mg ml −1 of OVA-alexa fluor 647 for 2.5 h at either 4 °C (4 deg) or 37 °C (37 deg). Antigen uptake was then measured by flow cytometry; N =7. ( d ) CCR7 expression by WT and KI BMDCs was determined by flow cytometry, with representative histogram (WT solid line; KI dashed line; isotype control shaded line) and pooled data from N =3. ( e ) Venn diagram showing numbers and overlap of the gene expression profiles of in vivo migratory DCs [29] and KI GM-CSF-cultured BMDCs. Significant values in ( c , d ) were calculated using the Student’s t -test, and the P -value in ( e ) was calculated by Hypergeometric test. All P -values are shown as <0.05*, <0.01**. Full size image Crucially, CCR7, which is essential for DC migration to lymph nodes, was found to be significantly upregulated in knock-in DCs, as determined by next-generation sequencing ( Fig. 3b ) and flow cytometry ( Fig. 3d ). By comparing gene expression profiles to previously described profiles of DC populations in vivo [29] , it became apparent that there was a significant overlap of the transcriptomes of knock-in DC and in vivo migratory DC populations (non-lymphoid tissue cDCs that have migrated to lymph nodes) ( Fig. 3e and Supplementary Dataset 3 ). In migratory DCs, beta2-integrins ( Itgb2 and Itgax genes) are downregulated, while CCR7 is upregulated; the same is true in knock-in DC (where beta2-integrins also display reduced adhesiveness due to the TTT/AAA mutation). Functional annotational clustering analysis [30] of genes that were upregulated in both migratory and knock-in DCs further ( Supplementary Data set 3 ) revealed that genes encoding for proteins involved in small GTPase signal transduction (such as Arhgef40, Rabgap1l, Net1, Rap2b), zinc-finger containing proteins (Cbl-b, Trim24 etc) and certain cell adhesion proteins (VCAM-1) were common to both types of cells. In contrast, genes encoding for proteins of certain other cellular pathways, such as macromolecule catabolic processes (some ubiquitin ligases and caspases), were not upregulated in KI DCs but were upregulated in migratory cells. Of the genes that were upregulated in both migratory and KI DCs, small GTPases such as Rap2 and cell adhesion proteins such as VCAM-1 are well known to regulate cell migration, and Cbl-b has been previously described as a negative regulator of beta2-integrin-mediated adhesion [31] . Therefore, it appears that the non-adherent knock-in DCs had switched on a transcriptional programme characteristic of DC populations that have matured and migrated to lymph nodes. Thus, the integrin-kindlin link, which is essential for DC adhesion to the environment, is crucial for restricting the DC maturation programme. To investigate whether switching on a transcriptional programme characteristic of migratory DCs influenced knock-in DC behaviour in vivo , we investigated numbers of DCs in lymphoid organs in beta2 TTT/AAA -integrin knock-in mice. We found that there were indeed significantly increased numbers of CD11c+ MHC class II+ DCs in the spleen and peripheral lymph nodes of knock-in animals compared with WT controls ( Fig. 4a ). Specifically, numbers of migratory CD11b+ and CD103+ DCs were increased in knock-in lymphoid tissues, whereas numbers of CD8+ and CD8− resident DCs were unaffected by the TTT/AAA mutation ( Fig. 4b ). T- and B-cell numbers in lymph nodes were normal in naive knock-in mice [1] and in immunized mice ( Fig. 4c ), but DC numbers in lymph nodes were increased in both resting and immunized knock-in mice ( Fig. 4d ). In addition, knock-in splenic DCs from both resting and immunized mice displayed significantly increased expression of CD86 in vivo , and a trend towards elevated CD40 expression, although this did not reach statistical significance ( Fig. 4e ). Importantly, following administration of fluorescent OVA antigen into the skin, we found increased numbers of OVA+ DCs in the draining lymph nodes 24 h later ( Fig. 4f ). Therefore, loss of the beta2-integrin-kindlin-3 link in DCs induces a switch to a mature phenotype in vitro and in vivo , and induced DC migration to lymph nodes and/or increased survival of KI DCs. 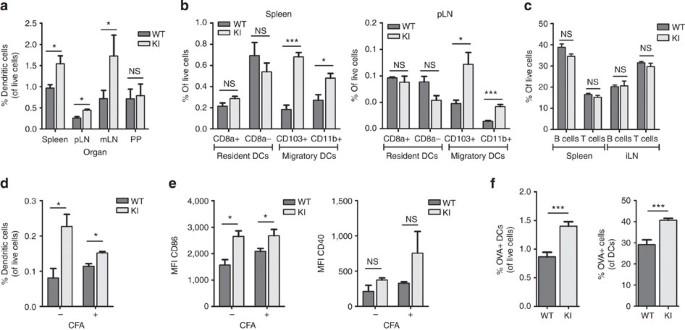Figure 4: Beta2-integrin knock-in DCs have a mature migratory phenotypein vivo. (a) Numbers of CD11c+ MHC class II+ DCs were quantified in lymphoid tissues of WT and KI mice by flow cytometry;N=4. (b) Resident and migratory DCs were quantified in WT and KI spleen and peripheral lymph nodes. Resident (CD8+ or CD8−) DCs were determined as CD3− CD19− B220− CD11c+ MHC class II+. Migratory DCs (CD103+ CD11b− or CD103− CD11b+) were identified as CD19− CD3− CD4− CD11c+ MHC class II+;N=5. (c) Percentages of CD19+ B cells and CD3+ T cells in the spleens and lymph nodes of CFA immunized mice 9 days post immunization; N=5. (d) Percentages of CD11c+ MHC class II+ DCs in lymph nodes of naive and CFA immunized mice 24 h post immunization;N=3. (e) Expression of CD86 and CD40 on total splenic DCs was examined in resting and CFA-immunized WT and KI mice 24 h post immunization;N=3. (f) WT and KI mice received OVA-alexa fluor 647 intracutaneously and 24 h later the draining lymph nodes were analysed for OVA+ DCs by flow cytometry;N=5. All error bars show s.e.m. and significant values were calculated using the Student’st-test. AllP-values are shown as <0.05*, <0.005***. Figure 4: Beta2-integrin knock-in DCs have a mature migratory phenotype in vivo . ( a ) Numbers of CD11c+ MHC class II+ DCs were quantified in lymphoid tissues of WT and KI mice by flow cytometry; N =4. ( b ) Resident and migratory DCs were quantified in WT and KI spleen and peripheral lymph nodes. Resident (CD8+ or CD8−) DCs were determined as CD3− CD19− B220− CD11c+ MHC class II+. Migratory DCs (CD103+ CD11b− or CD103− CD11b+) were identified as CD19− CD3− CD4− CD11c+ MHC class II+; N =5. ( c ) Percentages of CD19+ B cells and CD3+ T cells in the spleens and lymph nodes of CFA immunized mice 9 days post immunization; N=5. ( d ) Percentages of CD11c+ MHC class II+ DCs in lymph nodes of naive and CFA immunized mice 24 h post immunization; N =3. ( e ) Expression of CD86 and CD40 on total splenic DCs was examined in resting and CFA-immunized WT and KI mice 24 h post immunization; N =3. ( f ) WT and KI mice received OVA-alexa fluor 647 intracutaneously and 24 h later the draining lymph nodes were analysed for OVA+ DCs by flow cytometry; N =5. All error bars show s.e.m. and significant values were calculated using the Student’s t -test. All P -values are shown as <0.05*, <0.005***. Full size image Integrin-kindlin-actin links regulate DC maturation Maturation of DCs is well known to be associated with reduced adhesion and changes in cell morphology [32] , and we found that LPS maturation of DCs indeed significantly reduced adhesion to integrin ligands ( Fig. 5a ). To investigate whether loss of functional integrins was responsible for induction of DC maturation in beta2 TTT/AAA integrin knock-in cells, we analysed signalling and maturation status in beta2-integrin null DCs. Similar to the beta2 TTT/AAA integrin knock-in DCs, p-Syk and p-Akt levels were elevated in GM-CSF-stimulated beta2-integrin null DCs ( Fig. 5b ). These cells also expressed more MHC class II, CD80, CD86 and CD40 ( Fig. 5c ), and produced more IL-12p40 (in response to GM-CSF and LPS) and IL-10 (in response to LPS) than WT cells ( Fig. 5d ). These data indicate that the elevated signalling in knock-in DCs is due to the absence of functional beta2-integrins. 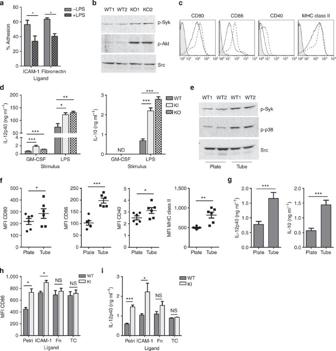Figure 5: Beta2-integrin-mediated ligand binding regulates DC maturation. (a) WT DCs were matured for 24 h by LPS stimulation and assessed for adhesion to ICAM-1 and fibronectin;N=3. (b) WT and beta2 null DC lysates were analysed for p-Syk, p-Akt and Src (loading control) by western blotting after 3 h GM-CSF stimulation. ShowsN=2, representative ofN=3. (c) Expression of CD80, CD86, CD40 and MHC class II by WT (solid line) and beta2 null (dashed line) DCs. Data are representative ofN=4 mice. Shaded line—isotype control. (d) Cytokine production by WT, KI and beta2 null (KO) DCs was measured after 24 h stimulation with 10 ng ml−1GM-CSF or 100 ng ml−1LPS;N=3. ND=not detectable. (e) WT DCs were adhered on plates or detached and placed in tubes and stimulated for 3 h with GM-CSF and analysed for GM-CSF receptor signalling by western blotting. ShowsN=2, representative of N=3. (f) WT DCs were adhered on plates or detached in tubes for 3 h before being stimulated with GM-CSF for a further 24 h. Expression of CD80, CD86, CD40 and MHC class II was then measured using flow cytometry;N=6. (g) IL-12p40 production by adhered and detached WT DCs in response to GM-CSF, and IL-10 production following LPS stimulation;N=6. (h,i) WT and KI BMDCs were placed on ICAM-1, fibronectin (Fn), non-treated petri dishes or tissue culture-treated plates (TC) for 3 h, and then stimulated with GM-CSF for a further 24 h. CD86 expression (h) and IL-12p40 production (i) were then measured;N=3. All error bars show s.e.m. and significant values were calculated using the Student’st-test. AllP-values are shown as <0.05*, <0.01**, <0.005***. Figure 5: Beta2-integrin-mediated ligand binding regulates DC maturation. ( a ) WT DCs were matured for 24 h by LPS stimulation and assessed for adhesion to ICAM-1 and fibronectin; N =3. ( b ) WT and beta2 null DC lysates were analysed for p-Syk, p-Akt and Src (loading control) by western blotting after 3 h GM-CSF stimulation. Shows N =2, representative of N =3. ( c ) Expression of CD80, CD86, CD40 and MHC class II by WT (solid line) and beta2 null (dashed line) DCs. Data are representative of N =4 mice. Shaded line—isotype control. ( d ) Cytokine production by WT, KI and beta2 null (KO) DCs was measured after 24 h stimulation with 10 ng ml −1 GM-CSF or 100 ng ml −1 LPS; N =3. ND=not detectable. ( e ) WT DCs were adhered on plates or detached and placed in tubes and stimulated for 3 h with GM-CSF and analysed for GM-CSF receptor signalling by western blotting. Shows N =2, representative of N=3. ( f ) WT DCs were adhered on plates or detached in tubes for 3 h before being stimulated with GM-CSF for a further 24 h. Expression of CD80, CD86, CD40 and MHC class II was then measured using flow cytometry; N =6. ( g ) IL-12p40 production by adhered and detached WT DCs in response to GM-CSF, and IL-10 production following LPS stimulation; N =6. ( h , i ) WT and KI BMDCs were placed on ICAM-1, fibronectin (Fn), non-treated petri dishes or tissue culture-treated plates (TC) for 3 h, and then stimulated with GM-CSF for a further 24 h. CD86 expression ( h ) and IL-12p40 production ( i ) were then measured; N =3. All error bars show s.e.m. and significant values were calculated using the Student’s t -test. All P -values are shown as <0.05*, <0.01**, <0.005***. Full size image We next directly assessed the role of integrin–ligand interactions in the regulation of signalling and maturation of DCs by comparing adhered WT DCs with WT DCs that were detached and placed in tubes. The results show that p-Syk and p-p38 levels were elevated in the detached cells compared with adhered cells ( Fig. 5e ). The expression of the co-stimulatory markers CD80, CD86, CD40 and MHC class II by WT DCs was significantly increased in detached cells compared with adhered cells when stimulated with GM-CSF ( Fig. 5f ). In addition, production of IL-12p40 and IL-10 was increased in detached cells compared with adhered cells following GM-CSF and LPS stimulation, respectively ( Fig. 5g ). Together, these results indicate that beta2-integrin-mediated ligand binding regulates signalling and maturation in myeloid DCs. To confirm this, we investigated IL-12 production ( Fig. 5h ) and CD86 expression ( Fig. 5i ) by WT and knock-in DCs plated on different substrates, for example, beta2-integrin substrates (petri dishes and ICAM-1), a beta1-integrin substrate (fibronectin) and tissue culture plates (unspecific substrate). As the knock-in mutation is in the beta2-integrin tail, knock-in DCs are not expected to display any abnormality when plated on a beta1-integrin substrate. Indeed, knock-in cells on beta2-integrin substrates displayed elevated maturation, while knock-in DCs on beta1-integrin substrates displayed similar activation to WT cells ( Fig. 5h,i ). These results indicate that WT beta2-integrin-mediated ligand binding and/or ligand-reinforced integrin tail interactions provides suppressory signals to the GM-CSF receptor complex, which are lost in KI DCs, and that ligand-induced beta1-integrin-mediated signals can compensate for the deficiency in function of beta2-integrins in KI cells. To directly assess the role of adhesion (rather than integrin-kindlin-3 contacts) in regulation of DC signalling, we further investigated whether Mn 2+ , a traditional extracellular activator of integrin-mediated adhesion, could rescue KI DC adhesion and at the same time suppress signalling. Although Mn 2+ treatment of cells did not result in a formal rescue of adhesion, low amounts of Mn 2+ did result in a slight increase in KI DC adhesion to ICAM-1 and iC3b ( Supplementary Fig. 5A ), but IL-12 production and CD86 expression were increased rather than decreased after Mn 2+ treatment ( Supplementary Fig. 5B ). These results show that increased adhesion alone, without integrin/kindlin links, was not sufficient to reduce GM-CSF receptor signalling in cells; rather, the integrin/kindlin link is required for integrins to suppress GM-CSF receptor signalling in DCs. The cortical actin cytoskeleton is known to restrict receptor movement and signalling in immune cells [21] . Integrin cytoplasmic domains are important in linking the plasma membrane to the actin cytoskeleton, and therefore play pivotal roles in actin organization. In addition, the integrin TTT/AAA mutation significantly perturbs integrin-mediated actin reorganization in cells [1] , [14] . Therefore, we investigated the subcellular localization of the beta2-integrins, kindlin-3 and the GM-CSF receptor in DCs. A significant amount of beta2-integrin, kindlin-3, talin and the GM-CSF receptor was localized to the cytoskeletal fraction of WT DCs, but the TTT/AAA-mutation of the integrin abolished these associations ( Fig. 6a ), indicating that the integrin-kindlin link is essential for actin recruitment of beta2-integrins and cytokine receptors. Levels of another membrane receptor, CD9, (a tetraspanin which mediates MHC II lateral associations in DCs [33] ) were equivalent in WT and knock-in cytoskeletal fractions ( Fig. 6a ), indicating that not all cell surface receptors are regulated in this way. To test whether the loss of the integrin-actin link is responsible for the increased signalling in knock-in DCs, cells were treated with cytochalasin D to disrupt actin filaments. Cytochalasin D treatment of WT DCs resulted in upregulation of p-Syk and p-MAPK ( Fig. 6b ), as well as an increase in CD86 and CD40 expression ( Fig. 6c ), and in IL-12p40 production ( Fig. 6d ). Together, these data indicate that ligand-reinforced integrin–actin interactions, regulated through kindlin-3, are necessary for the regulation of GM-CSF receptor signalling in DCs, and for the regulation of downstream effects including DC maturation. 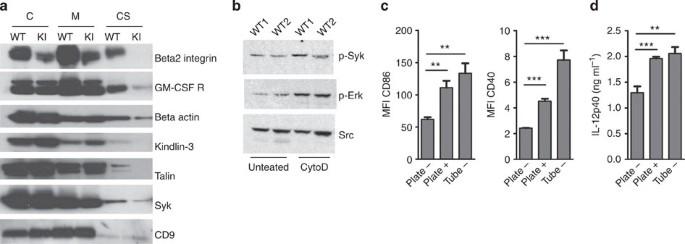Figure 6: Integrin-kindlin-actin links regulate DC maturation. (a) DC lysates were separated into subcellular fractions using a commercial kit (Thermo Scientific), as described in the Methods section, and then analysed by western blotting. C=cytoplasmic, M=membrane, CS=cytoskeleton. ShowsN=1 and is representative ofN=4. (b) p-Syk, p-Erk and Src (loading control) levels in lysates from WT DCs stimulated with GM-CSF, either untreated or treated with 10 μg ml−1cytochalasin D (CytoD).N=2 is shown, and is representative ofN=3. (c) WT DC expression of CD86 and CD40 in plates and tubes, with treatment with CytoD;N=4. (d) IL-12p40 production by WT DCs in plates and tubes, with CytoD treatment, following GM-CSF stimulation;N=4. Error bars show s.e.m. The Student’st-test was used to calculateP-values. Figure 6: Integrin-kindlin-actin links regulate DC maturation. ( a ) DC lysates were separated into subcellular fractions using a commercial kit (Thermo Scientific), as described in the Methods section, and then analysed by western blotting. C=cytoplasmic, M=membrane, CS=cytoskeleton. Shows N =1 and is representative of N =4. ( b ) p-Syk, p-Erk and Src (loading control) levels in lysates from WT DCs stimulated with GM-CSF, either untreated or treated with 10 μg ml −1 cytochalasin D (CytoD). N =2 is shown, and is representative of N =3. ( c ) WT DC expression of CD86 and CD40 in plates and tubes, with treatment with CytoD; N =4. ( d ) IL-12p40 production by WT DCs in plates and tubes, with CytoD treatment, following GM-CSF stimulation; N =4. Error bars show s.e.m. The Student’s t -test was used to calculate P -values. Full size image Syk is partly responsible for the mature DC phenotype Levels of p-Syk were elevated in beta2 TTT/AAA -integrin knock-in DCs ( Fig. 2f ). To investigate the role of Syk in the elevated DC activation status, we made use of the selective Syk inhibitor II [34] and a p38 inhibitor (SB203580). Syk inhibition of WT DCs in suspension resulted in a reduction of both co-stimulatory marker expression ( Fig. 7a ) and cytokine production ( Fig. 7b ), confirming that these activation properties of DCs are controlled by GM-CSF-induced Syk activity. Meanwhile, p38 inhibition in WT DCs reduced CD80 expression levels ( Fig. 7a ) and IL-10 production ( Fig. 7b ), but not CD86, CD40, MHC class II or IL-12p40 ( Fig. 7a,b ), suggesting that the p38 signalling pathway downstream of Syk regulates CD80 and IL-10 in GM-CSF-stimulated DCs. In addition, Syk inhibition in both beta2-integrin knock-in and null DCs resulted in a partial reduction of IL-12p40 and IL-10 production ( Fig. 7c ), showing that the active phenotype of knock-in DCs is due, in part, to elevated Syk activity. Together, these results reveal that integrin/kindlin-mediated signals negatively regulates downstream GM-CSF receptor signalling in DCs, mediated through Syk, which in turn regulates the expression of co-stimulatory molecules and production of cytokines. 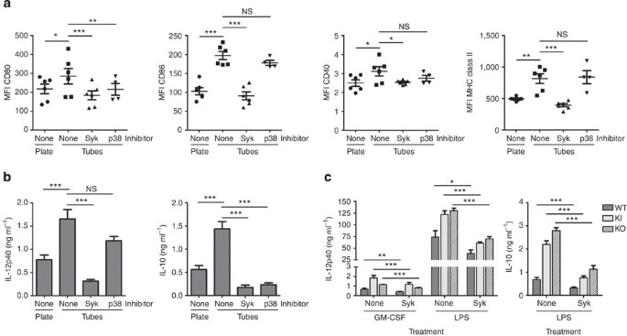Figure 7: Syk is partly responsible for the mature DC phenotype. (a,b) WT and KI BMDCs were put in plates or tubes and pre-treated with Syk and p38 inhibitors for 30 min before the addition of 10 ng ml−1GM-CSF or 100 ng ml−1LPS for 24 h. Expression of CD80, CD86, CD40 and MHC class II was then analysed by flow cytometry,N=4–6 (a). Levels of IL-12p40 and IL-10 were measured in culture supernatants after GM-CSF (for IL-12p40) or LPS (for IL-10) stimulation;N=4–6. (c) WT, KI and beta2 null (KO) DCs were pre-treated with Syk inhibitor II for 30 min, and then stimulated with GM-CSF (for IL-12p40) or LPS (for IL-10) for 24 h;N=3. ND=not detectable. In all cases error bars show s.e.m.. The Student’st-test was used to calculateP-values. AllP-values are shown as <0.05*, <0.01**, <0.005***. Figure 7: Syk is partly responsible for the mature DC phenotype. ( a , b ) WT and KI BMDCs were put in plates or tubes and pre-treated with Syk and p38 inhibitors for 30 min before the addition of 10 ng ml −1 GM-CSF or 100 ng ml −1 LPS for 24 h. Expression of CD80, CD86, CD40 and MHC class II was then analysed by flow cytometry, N =4–6 ( a ). Levels of IL-12p40 and IL-10 were measured in culture supernatants after GM-CSF (for IL-12p40) or LPS (for IL-10) stimulation; N =4–6. ( c ) WT, KI and beta2 null (KO) DCs were pre-treated with Syk inhibitor II for 30 min, and then stimulated with GM-CSF (for IL-12p40) or LPS (for IL-10) for 24 h; N =3. ND=not detectable. In all cases error bars show s.e.m.. The Student’s t -test was used to calculate P -values. All P -values are shown as <0.05*, <0.01**, <0.005***. Full size image Beta2-integrin knock-in DCs induce elevated Th1 responses ‘Muted’ DC activation has been associated with Th2 responses, while conventionally matured (TLR-activated) DCs generally promote Th1/Th17 responses [35] . In addition, Syk signalling in DCs is essential for Th1/Th17 responses in vivo [36] , [37] To investigate whether beta2 TTT/AAA integrin knock-in DCs specifically induce Th1/Th17 responses in vivo , WT or knock-in DCs were loaded with antigens that have previously been shown to promote differential T-helper cell subset polarization following DC adoptive transfer [38] ; the Th2 schistosome soluble egg antigen (SEA) and heat-killed Propionibacterium acnes that drives Th1/Th17 responses ( Supplementary Fig. 6A,B ). Beta2 TTT/AAA integrin knock-in DCs induced greater antigen-specific IFNγ production by T cells in both immunization groups ( Fig. 8a ), indicative of a stronger Th1 response. Conversely, the Th2 response (identified by IL-4, IL-5, IL-13 and IL-10) was significantly lower in the knock-in DC immunization groups, especially for the SEA group, which promoted the largest Th2 response ( Fig. 8a ). IL-17, indicative of a Th17 response, was only produced at marked levels in the P. acnes antigen group, where production was equivalent in the WT and knock-in DC immunization groups ( Fig. 8a ). Polyclonal stimulation confirmed the increased Th1 priming and impaired Th2 responses ( Supplementary Fig. 6C ). 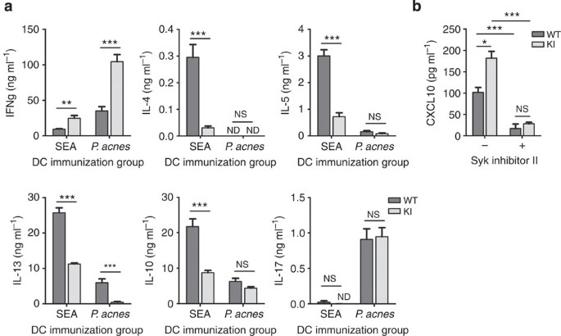Figure 8: Beta2-integrin knock-in DCs induce elevated Th1 responses. (a) WT or KI DCs were loaded with SEA or heat-killedP. acnesbefore being transferred into WT recipient mice subcutaneously into the foot. On day 7, the popliteal (draining) lymph nodes were removed, and the T-cell response analysed by measuring cytokine production followingin vitrorestimulation with antigen. Presented data are from one experiment, and is representative of two independent experiments, with five mice per group per experiment. (b) CXCL10 production was measured after 24 h stimulation of WT and KI DCs in the presence or absence of the Syk inhibitor;N=4. In all cases, error bars indicate s.e.m.. The Student’st-test was used to calculateP-values. NS=not significant. ND=not detectable. AllP-values are shown as <0.05*, <0.01**, <0.005***. Figure 8: Beta2-integrin knock-in DCs induce elevated Th1 responses. ( a ) WT or KI DCs were loaded with SEA or heat-killed P. acnes before being transferred into WT recipient mice subcutaneously into the foot. On day 7, the popliteal (draining) lymph nodes were removed, and the T-cell response analysed by measuring cytokine production following in vitro restimulation with antigen. Presented data are from one experiment, and is representative of two independent experiments, with five mice per group per experiment. ( b ) CXCL10 production was measured after 24 h stimulation of WT and KI DCs in the presence or absence of the Syk inhibitor; N =4. In all cases, error bars indicate s.e.m.. The Student’s t -test was used to calculate P -values. NS=not significant. ND=not detectable. All P -values are shown as <0.05*, <0.01**, <0.005***. Full size image We found increased production of CXCL10, a chemokine that promotes Th1 cell differentiation [39] , by knock-in DCs compared with WT DCs ( Fig. 8b ), which, together with the increased IL-12 production by these cells, may account for the elevated priming of Th1 responses by knock-in DCs in vivo . These data therefore demonstrate that beta2 TTT/AAA integrin knock-in DCs, which show increased signalling and an elevated activation state associated with migratory DCs, specifically promote elevated Th1 responses, and are strikingly impaired in their priming of Th2 responses, in vivo. In conclusion, we show that specific ligand-reinforced integrin tail interactions and integrin-mediated cytoskeletal organization play an unexpected role in restricting myeloid cell signalling and activation, and the maturation programme characteristic of migratory DCs, thereby regulating T-cell immune responses in vivo . Beta2-integrins are emerging as important negative regulators of immune-cell signalling, especially in myeloid cells, in stark contrast to the mainly positive role that integrins play in growth factor receptor signalling in other cell types. As such, beta2-integrins have been described to negatively regulate TLR and interferon signalling in macrophages [11] , [12] . In addition, active beta2-integrins in DCs and macrophages inhibit their priming of T cells [7] . Mechanisms by which beta2-integrins negatively regulate signalling are emerging. CD11b-induced Syk activation has been proposed as a mechanism to negatively regulate TLR signalling in macrophages [11] , and indirect mechanisms involving the signalling inhibitor A20 and the anti-inflammatory cytokine IL-10 have also been described [12] . However, the CD11b-integrin has also recently been reported to instead positively regulate TLR4 signalling in endosomes in DCs (as opposed to macrophages), and to be required for TLR4-triggered responses in vivo [13] . In contrast, in this study, we describe that ligand-reinforced beta2-integrin tail interactions with kindlin-3 and cytoskeletal coupling negatively regulate DC maturation through restricting GM-CSF receptor signalling. Therefore, in DCs, ablating beta2-integrin-mediated cytoskeletal organization (through mutation of the kindlin-binding site in the integrin, or beta2-integrins themselves) results in a strikingly different phenotype than ablating the CD11b integrin subunit alone, likely reflecting redundancy between different beta2-integrins in DCs, as DCs express (at least) CD11a- and CD11c-chains in addition to CD11b. Interestingly, we found that the integrin/kindlin connection also restricts GM-CSF receptor signalling in neutrophils. Neutrophilia is a significant symptom in murine models with defects in adhesion molecules [1] , [24] , [25] , [26] , [27] ; our data suggest that increased GM-CSF receptor signalling in these cells may contribute to the significant neutrophilia found in these mouse models. Intriguingly, ablating the beta2-integrin/kindlin-3 interaction results in DC maturation to a migratory phenotype, increased DC trafficking to lymph nodes and increased T-cell priming in vivo . Reprogramming of DCs to a mature, migratory phenotype by loss of integrin/kindlin links implies that beta2-integrins contribute to immune homeostasis by restricting DC maturation in tissues until migration and maturation is required. Does loss of ligand-induced integrin signals contribute to DC maturation/migration also under physiological conditions? Interestingly, migratory DCs found in lymph nodes express less beta2-integrins than their tissue counterparts ( Supplementary Data set 3 ) [29] , indicating that under steady-state conditions, beta2-integrins are indeed downregulated when cells migrate to lymph nodes, possibly through a cell-intrinsic effect during the DC life cycle. We speculate that beta2-integrins, which are not required for DC migration to lymph nodes in steady state [6] , instead mediate DC interactions with their extracellular environment in peripheral tissues, which restricts their migration to lymph nodes. Loss of ligand-binding due to integrin downregulation reprogrammes DCs and contributes to migration to lymph nodes under steady-state conditions. In addition, it is well described that during DC maturation due to external stimuli, such as TLR stimulation, adhesion is downregulated and the cell morphology and actin cytoskeleton are fundamentally altered [32] , [40] , and the cells become more migratory [40] , and we show here that adhesion to integrin-ligands is indeed reduced in LPS-matured DCs. Therefore, maturation-induced loss of ligand-binding and/or cytoskeletal coupling may promote DCs to switch on the transcriptional programme that allows for their migration to lymph nodes and for the subsequent activation of T cells. The elevated maturation status in DCs lacking beta2-integrin-mediated cytoskeletal organization was mediated by increased GM-CSF receptor signalling. The membrane skeleton is essential for controlling signalling in resting immune cells [21] , [41] and integrins act as links or integrators between the cell exterior and the cell cytoskeleton in cells [42] . They would therefore be well positioned for forming ‘pickets’ in the ‘picket-fence’ model of the plasma membrane and for restricting movement of receptors in the plasma membrane [43] . We propose that ligand-reinforced integrin-kindlin linkages fundamentally restrict the movement of the actin-linked GM-CSF receptor (and possibly other receptors or adapter proteins) at the DC plasma membrane, thereby limiting downstream signalling, a function of integrins in immune cells that has not previously been appreciated ( Supplementary Fig. 8 ). We further show that increased GM-CSF receptor-induced Syk signalling is, in part, responsible for the elevated activation phenotype in these knock-in DCs. TLR responses were also elevated in knock-in DCs, although TLR signalling did not further activate Syk in these cells. Interestingly, a complex between the beta-common chain of IL-3/IL-5/GM-CSF receptors and the ITAM-containing Fc receptor γ-chain has been previously described, leading to recruitment of Syk to the IL-3 receptor in basophils [23] ; a similar mechanism may be at play in DCs and neutrophils. The exact mechanism(s) of integrin-mediated regulation of signalling receptors in DCs need to be established in future studies. A striking result from this work was that beta2 TTT/AAA -integrin knock-in DCs, which displayed an elevated activation state, induced elevated Th1 responses in vivo , while Th2 priming was impaired. Indeed, highly activated DCs have previously been described to preferentially promote a Th1 response [44] , while Th2 responses are generally associated with a ‘muted’ DC activation state [35] . In addition, Syk signalling in DCs has been previously reported to be essential for Th1 responses in vivo [36] , [37] . We show that increased Syk signalling resulted in elevated DC activation and increased IL-12 production by knock-in DCs, which may explain why these cells were poised to induce Th1, rather than Th2, immune responses in vivo , through counter-regulation of Th2 activation. In contrast, other Th1 polarizing factors, such as CD70 [45] , although more highly expressed in knock-in DCs, were expressed at very low levels and therefore were unlikely to contribute to the Th1 polarization by the knock-in DCs. Also, IRF4, a transcription factor in DCs that has recently been described to be essential for Th2 development [46] , was not different between WT and knock-in cells. However, the GM-CSF-cultured knock-in DCs produced more CXCL10, a chemokine which has been shown to be involved in DC-dependent Th1 responses in vivo [39] ; CXCL10 production was also dependent on Syk. Th17 priming by the knock-in DCs was normal, likely reflecting the observation that production of IL-6, the key cytokine that drives Th17 differentiation in this model [47] , was minimally affected by the knock-in mutation. Beta2-integrins have been shown to promote tolerance [10] , suppress colitis and dermatitis [48] , [49] and protect against endotoxic shock [11] , consistent with regulatory and homeostatic roles of these integrins in immune responses in vivo . In addition, autoimmune colitis has been reported in several LAD-I patients, further supporting the notion that the absence of beta2-integrin-mediated function in vivo results in unregulated immune responses [50] , [51] , [52] . Beta2-integrins, therefore, play dual roles in the immune system as they influence both the recruitment of leukocytes to sites of inflammation, as well as the regulation of inflammatory responses by restricting signalling in myeloid cells when they interact with their environment. Our report has unravelled novel roles of beta2-integrins in immune-cell functions, and has demonstrated that the beta2-integrin-kindlin-3 interaction, in addition to regulating T-cell adhesion and homing [1] , also plays an unexpected role in restricting GM-CSF-induced Syk signalling, the transcriptional programme characteristic of mature migratory DCs, and in regulating Th1/Th2 immune responses. Our results therefore expand on current models of how beta2-integrins regulate immune homeostasis. In addition, the induction of a migratory DC phenotype by targeting beta2-integrins may be of use in the design of more effective dendritic cell-based immunotherapies. Mice Mice were maintained in the Wellcome Trust Biocentre at the University of Dundee, the School of Biological Sciences, University of Edinburgh, or the University of Helsinki, Finland, in compliance with UK Home Office Animals (Scientific Procedures) Act 1986 and the Finnish Act on Animal Experimentation (62/2006), respectively. Animal experiments were approved by the Home office (UK) and the national Animal Experiment Board (Finland), respectively. We have previously generated the Itgb2 knock-in mice [1] . C57Bl/6 mice were obtained from Charles River and beta2 null mice from JAX (catalogue number 003329). Age- and sex-matched male or female mice aged 8–12 weeks were used in experiments. Leukocyte isolation and culture preparation DCs were generated by culturing bone marrow for 10 days in 10 ng ml −1 GM-CSF (Peprotech), with feeding on days 3, 6 and 8. Alternatively, bone marrow cells were cultured in 200 ng ml −1 Flt3 ligand (ImmunoTools) for 8 days, with feeding on day 4. Macrophages were generated by culture of bone marrow cells in M-CSF (Peprotech) for 7 days, with feeding on day 3. Non-treated tissue culture plates were used for all cultures. Neutrophils were isolated from bone marrow by negative selection using microbeads (Miltenyi Biotec) according to the manufacturer’s instructions. Neutrophil survival in vitro in GM-CSF was determined by duplicate Trypan blue counts after 44 h of culture. Reagents Syk inhibitor II (Calbiochem, CA, USA) and p38 inhibitor (SB203580, Cell Signaling) were used at 10 μM. Cytochalasin D (Calbiochem, CA, USA) was used at 10 μg ml −1 . Bafilomycin (Sigma-Aldrich, MO, USA) was used at 12.5 nM. IL-3 (R&D systems) was used at the concentrations indicated in the figure. Integrin ligands ICAM-1 (R&D systems) and Fibronectin (Calbiochem) were coated onto cell culture plates at 3 and 5 μg ml −1 , respectively, by incubation at 4 °C overnight. Static adhesion assays ICAM-1 (6 μg ml −1 , R&D Systems, MN, USA) or iC3b (1 μg ml −1 , R&D Systems, MN, USA) were coated in duplicate/triplicate onto flat-bottomed 96-well Maxisorp plates (Nunc) overnight at 4 °C. Wells were blocked with 3% human serum albumin for 1 h 15 min at 37 °C. DCs were resuspended at 2 × 10 6 cells ml −1 in binding medium (RPMI plus 0.1% bovine serum albumin, 40 mM Hepes and 2 mM MgCl 2 ) and stimulated, where indicated, with 200 nM PdBu (Sigma-Aldrich, MO, USA). Cells were allowed to adhere for 20 min before gentle washing and detection as in ref. 53 . Priming assays DCs were activated with 100 ng ml −1 LPS (Sigma-Aldrich, MO, USA) overnight and loaded with 1 μM ovalbumin peptide 323–339 (AnaSpec, CA, USA) for 90 min. After washing, DCs were cultured with purified CD4 OT-II T cells at a ratio of 1:10. Moloney murine leukaemia virus H19env peptide 123–141 was emulsified in complete Freund’s adjuvant (CFA, Sigma-Aldrich, MO, USA) using a sonicator. Mice were immunized with a total of 100 μg peptide/CFA subcutaneously into the hind legs. Alternatively, DCs were activated with 100 ng ml −1 LPS (Sigma-Aldrich, MO, USA) overnight and loaded with 50 μg ml −1 H19env peptide for 90 min. A total of 1–2 × 10 6 LPS-activated peptide-loaded DCs were injected intravenously into mice. DCs were loaded with 25 μg ml −1 Schistosomal egg antigen (SEA, in-house) or 10 μg ml −1 heat-killed Propionibacterium acnes (in-house) overnight. A total of 5 × 10 5 cells were injected into the feet of recipient C57Bl/6 mice. Seven days post immunization, popliteal (draining) lymph nodes were extracted, and cells restimulated with antigens (15 μg ml −1 SEA, 1 μg ml −1 heat-killed P. acnes , plate-bound anti-CD3 (clone 2C11)) in vitro for 72 h. Supernatants were taken and cytokine production analysed by ELISA using paired antibody kits (ebioscience) according to standard protocols. Antigen uptake assays For in vitro antigen uptake by BMDCs, cells were cultured with 0.1 mg ml −1 OVA-alexa fluor 647 (Life Technologies) for 2.5 h at either 4 or 37 °C. To assess in vivo antigen uptake by DCs and migration to lymph nodes, mice were shaved, tape stripped three times and 50 μg OVA-alexa fluor 647 injected intracutaneously. After 24 h, draining lymph nodes were removed, and DC antigen uptake analysed by flow cytometry. Optical trapping DC-T-cell interaction forces were measured using a custom optical trapping system (Glass et al , manuscript in preparation). The beam from a Ventus IR, 3 W, continuous wave laser (Laser Quantum, UK) at a wavelength of 1,064 nm was expanded to just overfill a Spatial Light Modulator (SLM; Boulder Nonlinear Systems, CO, USA). The SLM consisted of 512 × 512 individually addressable pixels, altering the phase of the light and projecting a hologram onto the back aperture of the microscope objective. Holograms were calculated and displayed on the SLM using the ‘Red Tweezers’ software [54] (University of Glasgow), providing flexibility to alter the position of a triple-spot optical trap within the field-of-view and adjust the trap positions relative to each other to reflect the individual cell size. The triple-spot laser beam was directed into a Nikon TE2000-U inverted fluorescence microscope (Nikon, UK). The optical tweezers were calibrated with the laser beam power using the escape force method [54] . For initial contact force measurement, DCs were seeded into an Ibidi μ-slide VI 0.4 (Ibidi, Germany) and purified OT-II T cells added. A single T cell was optically trapped, brought into contact with a DC, and the shutter was immediately closed. After 2 min, the trapping laser was unblocked and the power of the beam increased in increments until the T cell was separated from the DC, at which point the force of the trap was taken to be equal to the interaction force. For quantifying DC–T-cell interactions after 24 h, cells were incubated in an Ibidi μ-slide 8-well before cell pairs were identified. Measurements were taken as described above. Flow cytometry and tetramer staining For ex vivo analysis of DCs in lymphoid tissues, organs were digested in 1 mg ml −1 collagenase type II (Life Technologies) with 2 mM EDTA for 20–30 min at room temperature with agitation. Tetramer staining was performed in 96-well round-bottom plates. PE-labelled MHC class II tetramers (NIH tetramer core facility, USA) containing either the H19env peptide or an irrelevant peptide control were used at 1/100 dilution in RPMI plus 10% fetal bovine serum, for 3 h at 37 °C. The following conjugated antibodies were used (all ebioscience, unless otherwise stated): CD18 (C71/16), CD11a (2D7), CD11b (M1/70), CD11c (HL3), CD80 (16-10A1), CD86 (GL1), CD40 (3/23), MHC class II (M5/114.15.2), CD103 (2E7), CD69 (H1.2F3), CD25 (PC61), CD44 (IM7), CD3 (145-2C11), CD4 (RM4-5), CD8a (53-6.7), CD19 (1D3), B220 (RA3-6B2), F4-80 (BM8), Gr-1 (RB6-8C5), CCR7 (4B12), GM-CSF receptor beta-common chain (K-17, Santa Cruz Biotech). All FITC-conjugated antibodies were used at 1:100 dilution, and all other antibodies were used at 1:200 dilution. Fc block (clone 2.4G2, BD Biosciences, 1:100 dilution) was included in all stains. Propidium iodide or DAPI (Sigma) was added immediately before acquisition on an LSR Fortessa flow cytometer (Becton Dickinson). Data were analysed using FlowJo software (TreeStar, OR, USA). Immunoblotting DCs were lysed in 1% Tx-100, 150 mM NaCl, 50 mM Tris pH 7.4, 10 mM ethylenediamine tetraacetic acid (EDTA), 50 mM NaF and 1 mM sodium orthovanadate, containing protease inhibitor cocktail (Roche). Alternatively, DCs were fractionated into subcellular fractions using a subcellular protein fraction kit (Thermo Scientific, NH, USA) according to the manufacturer’s instructions. Primary antibodies against the following proteins were used (Cell Signaling, unless otherwise stated): p-JAK2, p-STAT5, p-Syk, p-p38, p-Erk, p-Akt, Akt, Src, Syk, beta-actin, beta2-integrin (Abcam, MA, USA), GM-CSF receptor beta-common chain (Santa Cruz Biotechnology, CA, USA), kindlin-3 (Sigma-Aldrich, MO, USA), talin, CD9 (BD Biosciences). After incubation in horseradish peroxidase–conjugated secondary antibodies, blots were developed by standard chemiluminescence techniques. All uncropped blots are shown in Supplementary Fig. 7 . RNA preparation and next-generation sequencing RNA was prepared from DCs cultured from three WT and three knock-in mice using the NucleoSpin RNA II kit (Macherey-Nagel). RNA samples were analysed by the Finnish Microarray and Sequencing Centre (Turku, Finland) after the quality of RNA was checked using the Bioanalyser (Agilent). Sequencing of samples was performed on the Illumina HiSeq2500 using 1 × 50 bp runs on single-end libraries. Selection of differentially expressed genes All Sequencing data in the fastq format were analysed using the Chipster General User Interface [55] . Sequences were trimmed at the 5′end (minimum score 20) and filtered with a maximum length of 50 bp using PRINSEQ [56] . Reads were aligned using TopHat2 [57] onto the Mouse genome (mm10) for each sample (total genes 37 315) and the aligned reads per gene were counted using HTseq. Differential expression analysis was performed by negative binomial distribution using edgeR [58] and DESeq [59] software. Common genes chosen by both these software packages were chosen and those genes that had an expression level of less than 10 RPKM (Reads per kilobase per million reads) in at least one of the upregulated samples were discarded. This left a total of 855 genes expressed higher in WT DCs and 862 genes expressed higher in knock-in DCs. Comparison with resident and migratory DCs Differentially expressed genes from migratory and resident DCs identified from a previous microarray study [29] were downloaded ( Supplementary Data set 3 ). Genes that were represented more than once through multiple Microarray probes were combined and genes without an ENSMUS number were removed. This left a total of 249 genes upregulated in migratory DCs and 93 genes upregulated in resident DCs. The identities of these genes were then compared with the list of differentially expressed genes from our study. Statistical analysis The Student’s 2-tailed t -test, Mann–Whitney U -test, ANOVA test (Graphpad Prism, CA, USA), and Hypergeometric test (GeneProf) were used to calculate statistical significance. All P -values are shown as *<0.05, **<0.01, ***<0.005. How to cite this article : Morrison, V. L. et al . Loss of beta2-integrin-mediated cytoskeletal linkage reprogrammes dendritic cells to a mature migratory phenotype. Nat. Commun. 5:5359 doi: 10.1038/ncomms6359 (2014).